Dissecting a central flip-flop circuit that integrates contradictory sensory cues inC. elegansfeeding regulation Feeding behaviour is modulated by both environmental cues and internal physiological states. Appetite is commonly boosted by the pleasant smell (or appearance) of food and destroyed by a bad taste. In reality, animals sense multiple environmental cues at the same time and it is not clear how these sensory inputs are integrated and a decision is made to regulate feeding behaviour accordingly. Here we show that feeding behaviour in Caenorhabditis elegans can be either facilitated by attractive odours or suppressed by repellents. By identifying mutants that are defective for sensory-mediated feeding regulation, we dissected a central flip-flop circuit that integrates two contradictory sensory inputs and generates bistable hormone output to regulate feeding behaviour. As feeding regulation is fundamental to animal survival, we speculate that the basic organizational logic identified here in C. elegans is likely convergent throughout different phyla. Animals must face complicated variations in their circumstances. These environmental factors include 'good' and 'bad' physical and chemical stimuli, such as pleasant and repulsive smells, and high and low temperatures. However, how these contradictory factors modulate behaviour is not clear. Caenorhabditis elegans is equipped with multiple sensory modalities that can detect environmental cues, including odours, tastes, osmolarity, temperature and mechanical touch. It can sense hundreds of water-soluble and volatile molecules, which can evoke distinct behaviours, such as attraction, avoidance, feeding or mating [1] . Two pairs of amphid sensory neurons, AWA and AWC, mediate chemotaxis to attractive volatile odorants [2] , whereas another pair of chemosensory neurons, ASH, mediate avoidance behaviour to high osmolarity, high concentration of volatile odours, bitter alkaloids (such as quinine) and detergents [3] , [4] , [5] . It is not clear how attractive and repellent sensory cues are integrated to regulate animal behaviour. C. elegans feeds via powerful pumping of the pharyngeal tube, which results in bacterial ingestion, concentration, grinding and forcing of the crushed suspension into the intestinal lumen [6] . Selecting rate of pumping as a readout and challenging C. elegans with attractants and repellents, we find that attractants and repellents facilitate and suppress feeding in C. elegans , respectively. Furthermore, by identifying and characterizing mutants that are defective in sensory-mediated feeding facilitation and suppression, we demonstrate a C. elegans molecular and neural circuit that integrates contradictory sensory inputs in the regulation of pumping rate. Rather than a linear summation of sensory stimuli, we reveal nonlinear integration at the central neurosecretory cells. We conclude that the 'winner takes all' feature of the central integration circuit ensures a stable feeding behaviour in the presence of noisy environmental cues. Sensory cues mediate feeding facilitation or suppression We first tested whether organisms as simple as worms can change their feeding behaviour in response to environmental cues, similar to human beings. We challenged worms with either attractive odorants, diacetyl and low concentrations of isoamylol [2] , or repellents, such as quinine and a high concentration of isoamylol [7] , [8] . We found that diacetyl concentrations of 10% or more increased the pumping rate by ~25%, a phenomenon we call feeding facilitation ( Fig. 1a ). Feeding facilitation was also observed for low concentrations of isoamylol (10 −4 to 10 −5 dilution, Supplementary Fig. S1 ), an attractant which is mainly detected by AWC neurons [2] . Moreover, we observed feeding suppression, in which pumping rates were decreased to a very low level, in a dose-dependent manner by high concentrations of isoamylol or quinine ( Fig. 1a,b ). On the basis of dose–response curves, we chose concentrations of 100, 100% and 5–10 mM for diacetyl, isoamylol and quinine, respectively, for subsequent experiments, unless otherwise stated. We measured pumping rates between 5 and 10 min, when the stimuli had their maximum effects ( Fig. 1c ). Possible influences of these chemicals on locomotion were excluded by monitoring body bends under short- or long-term chemical exposure ( Supplementary Fig. S2 ). 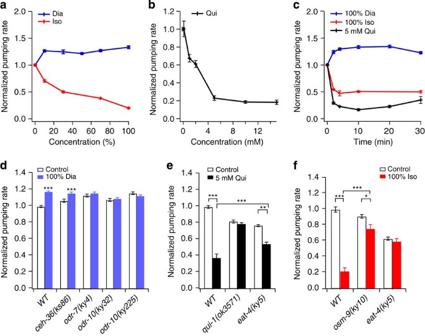Figure 1:C.elegansdisplays sensory-induced feeding facilitation and suppression. (a,b) Diacetyl, isoamylol and quinine modulate the pumping rate in a concentration-dependent manner. (c) Time courses of action of diacetyl, isoamylol and quinine on modulating pumping rate. (d) Diacetyl-induced feeding facilitation requires odour sensation through AWA neurons. The pumping rate of various strains was measured under the same conditions and normalized to that of wild-type (WT; N2) animals. Mutation of AWA diacetyl receptorodr-10and AWA developmental geneodr-7eliminated the enhancement of pumping rate induced by exposure to 100% diacetyl on food. (e) Quinine-induced feeding suppression requires ASH neurons through its receptor QUI-1 and glutamate signalling. Normalized pumping rates under control and 5 mM quinine feeding conditions are shown. (f) Isoamylol-induced feeding suppression requires ASH neurons through OSM-9 and glutamate signalling. Normalized pumping rates under control conditions and with exposure to 100% isoamylol in food are shown. Dia, diacetyl; Iso, isoamylol; Qui, quinine. The feeding rates of N2 animals used for normalization ina–fare 238, 248, 247, 250, 248 and 263 pumps per min, respectively. Statistics (d–f): *P<0.05, **P<0.01, ***P<0.001 (Student'st-test). Data are averaged from 10 to 12 animals for each condition. Error bars represent s.e.m. Figure 1: C.elegans displays sensory-induced feeding facilitation and suppression. ( a , b ) Diacetyl, isoamylol and quinine modulate the pumping rate in a concentration-dependent manner. ( c ) Time courses of action of diacetyl, isoamylol and quinine on modulating pumping rate. ( d ) Diacetyl-induced feeding facilitation requires odour sensation through AWA neurons. The pumping rate of various strains was measured under the same conditions and normalized to that of wild-type (WT; N2) animals. Mutation of AWA diacetyl receptor odr-10 and AWA developmental gene odr-7 eliminated the enhancement of pumping rate induced by exposure to 100% diacetyl on food. ( e ) Quinine-induced feeding suppression requires ASH neurons through its receptor QUI-1 and glutamate signalling. Normalized pumping rates under control and 5 mM quinine feeding conditions are shown. ( f ) Isoamylol-induced feeding suppression requires ASH neurons through OSM-9 and glutamate signalling. Normalized pumping rates under control conditions and with exposure to 100% isoamylol in food are shown. Dia, diacetyl; Iso, isoamylol; Qui, quinine. The feeding rates of N2 animals used for normalization in a–f are 238, 248, 247, 250, 248 and 263 pumps per min, respectively. Statistics ( d – f ): * P <0.05, ** P <0.01, *** P <0.001 (Student's t -test). Data are averaged from 10 to 12 animals for each condition. Error bars represent s.e.m. Full size image We next tried to understand how these modulations of feeding are achieved. It has been suggested that high concentrations of diacetyl can be detected by both AWA and AWC neurons [9] . We found that the stimulatory effect of 100% diacetyl on pumping was maintained in ceh-36 mutants, but abolished in odr-10 and odr-7 mutants ( Fig. 1d ), a defect which was fully rescued by introducing the odr-10 and odr-7 genomic transgenes, respectively ( Supplementary Figs S3,S4 ). The ceh-36 gene is required for the development and function of AWC neurons [10] , [11] , while the odr-10 gene is normally expressed exclusively in AWA neurons under the control of odr-7 and encodes a G-protein-coupled receptor that detects diacetyl [7] , [8] . These data indicate that diacetyl induces feeding facilitation mainly via sensing through the AWA sensory neurons. It should be noted that odr-10 and odr-7 mutants had elevated pumping rates compared with N2 animals in the absence of diacetyl, suggesting an involvement of AWA neurons in the regulation of basal pumping rate. It has been suggested that quinine is detected mainly by ASH neurons [8] . Quinine-mediated feeding suppression was completely abolished in the absence of qui-1 ( Fig. 1e ), which is required for ASH-mediated avoidance of bitter tastes [8] . It has been reported that high concentrations of volatile repellents are also detected by ASH neurons [5] . OSM-9, the worm homologue of the vertebrate nociceptive channel TRPV1 (the capsaicin receptor), generally participates in perception of repellents by ASH neurons [12] , [13] . In osm-9 mutants, the isoamylol avoidance index was greatly reduced ( Supplementary Fig. S5 ) and isoamylol-induced feeding suppression ( Fig. 1f ) was largely abolished. Quinine and isoamylol were still able to inhibit pumping in odr-10 and odr-7 mutants ( Supplementary Fig. S6 ), excluding the participation of these genes in feeding suppression. ASH neurons relay nociception via glutamatergic synapses. Both quinine- and isoamylol-mediated feeding suppressions were significantly decreased in eat-4 mutants, which are defective in glutamate transmission [14] . Expression of eat-4 genomic transgenes restored quinine-induced feeding suppression in eat-4 mutants ( Supplementary Fig. S7 ). Taken together, the above experiments confirm that feeding modulation mediated by different sensory modalities is conserved in C. elegans . Circuits underlying feeding facilitation We then explored the signalling pathways downstream of different sensory modalities. The neurotransmitter 5-hydroxytryptamine (5-HT, serotonin) regulates food-related behaviours and physiology in diverse vertebrate and invertebrate phyla [15] , [16] , [17] , [18] . It is known that 5-HT increases pumping rate in the absence of food [19] , while tph-1 mutants, which fail to synthesize 5-HT, display reduced feeding [17] . In the presence of food, it has been reported that exogenous 5-HT (13 mM) did not stimulate pumping [20] . In contrast, we observed ~25% increase in pumping rate on exogenous administration of 2 mM 5-HT ( Fig. 2a ), which is consistent with observations made in a study by Srinivasan et al ., [21] in which 5 mM 5-HT was used. Interestingly, we confirmed that only low concentrations of 5-HT (2–5 mM) could facilitate feeding in the presence of food ( Supplementary Fig. S8 ), suggesting that high concentrations of 5-HT might induce adaptation or autoinhibition in feeding regulation, as proposed by Hobson et al . [20] Diacetyl-mediated, but not 5-HT-mediated, enhancement of pumping was abolished in tph-1 mutants ( Fig. 2a,b ), suggesting the involvement of 5-HT in sensory-mediated feeding facilitation. In hermaphrodite C. elegans , tph-1 expression is limited to only a few serotonergic neurons, such as NSM, ADF and HSN [17] , [22] . To locate the release site of 5-HT, we used neuron-specific promoters to drive the expression of TPH-1 in tph-1 mutants. Reconstitution of tph-1 in a subset of cells that overlap with serotonergic neurons in the NSM rescued the feeding facilitation ( Fig. 2c ), suggesting that TPH-1 acts in NSM neurons. 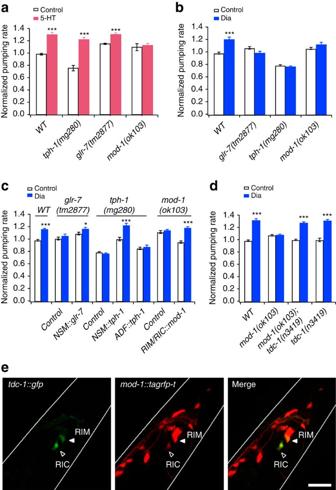Figure 2: Identification of the neurons and genes required for diacetyl (Dia)-induced feeding facilitation. (a) GLR-7 acts upstream of serotonin release, whereas MOD-1 acts downstream of serotonin. Serotonin (2 mM) was applied exogenously. (b) Diacetyl-induced feeding facilitation requiresglr-7,tph-1andmod-1, which encode an ionotropic glutamate receptor, an enzyme for making 5-HT, and a novel 5–HT-gated chloride channel, respectively. Normalized pumping rates for various strains under control and diacetyl (100%) stimulation conditions are shown. (c) Neuron-specific transgene rescue experiments localized the functional sites ofglr-7andtph-1to NSM andmod-1to RIM/RIC neurons. Promoters used werePsrh−142for ADF,Pceh−2for NSM in thetph-1rescue experiment,Ptph−1for NSM in theglr-7rescue experiment,Ptdc−1for RIM/RIC. (d) The loss-of-facilitation phenotype ofmod-1mutants was suppressed by eliminatingtdc-1, which is required for making tyramine.tdc-1itself is not required for feeding facilitation. (e) Expression patterns ofmod-1andtdc-1. MOD-1 and TDC-1 are coexpressed in RIM and RIC neurons. Scale bar, 20 μm. The feeding rates of N2 animals used for normalization ina–dwere 250, 253, 240 and 239 pumps per min, respectively. Statistics (a–d): *P<0.05 and ***P<0.001 (Student'st-test). Data are averaged from 10 to 12 animals for each condition. Error bars represent s.e.m. WT, wild type. Figure 2: Identification of the neurons and genes required for diacetyl (Dia)-induced feeding facilitation. ( a ) GLR-7 acts upstream of serotonin release, whereas MOD-1 acts downstream of serotonin. Serotonin (2 mM) was applied exogenously. ( b ) Diacetyl-induced feeding facilitation requires glr-7 , tph-1 and mod-1 , which encode an ionotropic glutamate receptor, an enzyme for making 5-HT, and a novel 5–HT-gated chloride channel, respectively. Normalized pumping rates for various strains under control and diacetyl (100%) stimulation conditions are shown. ( c ) Neuron-specific transgene rescue experiments localized the functional sites of glr-7 and tph-1 to NSM and mod-1 to RIM/RIC neurons. Promoters used were P srh−142 for ADF, P ceh−2 for NSM in the tph-1 rescue experiment, P tph−1 for NSM in the glr-7 rescue experiment, P tdc−1 for RIM/RIC. ( d ) The loss-of-facilitation phenotype of mod-1 mutants was suppressed by eliminating tdc-1 , which is required for making tyramine. tdc-1 itself is not required for feeding facilitation. ( e ) Expression patterns of mod-1 and tdc-1 . MOD-1 and TDC-1 are coexpressed in RIM and RIC neurons. Scale bar, 20 μm. The feeding rates of N2 animals used for normalization in a – d were 250, 253, 240 and 239 pumps per min, respectively. Statistics ( a – d ): * P <0.05 and *** P <0.001 (Student's t -test). Data are averaged from 10 to 12 animals for each condition. Error bars represent s.e.m. WT, wild type. Full size image We identified glr-7 in further screens for mutants with disrupted responses to diacetyl ( Fig. 2b ). glr-7 encodes a non- N -methyl- D -aspartate-type ionotropic glutamate receptor, and its exact function in C. elegans is unclear. Interestingly, we found that the glr-7 mutation abolished diacetyl-mediated, but not 5-HT-mediated, feeding facilitation ( Fig. 2a,b ), suggesting that GLR-7 acts upstream of 5-HT release. glr-7 is expressed in the pharyngeal neurons, including I1, I2, I3, I6, MI and NSM [23] . Expression of glr-7 under the control of its own promoter ( Supplementary Fig. S9 ) or NSM-specific promoter ( Fig. 2c ) rescued the defect in glr-7 mutants, suggesting that GLR-7 acts, at least partially, in NSM neurons to stimulate 5-HT release. The signal that triggers GLR-7 is likely from the I1, I2, I3 or MI neurons, which send chemical synapses to the NSM neurons. Of the C. elegans 5-HT receptors examined, we found that only MOD-1 was required for both diacetyl- and 5–HT-mediated feeding facilitation ( Fig. 2a,b,d , see also Table 1 ). MOD-1 is a novel 5–HT-gated chloride channel and is expressed in the AIA, AIB, AIY, AIZ and RID interneurons, as well as in a number of additional unidentified neurons in the head, ventral cord and tail [24] , [25] . MOD-1 has been suggested to function in regulating locomotion [24] , [25] , [26] , [27] and egg laying [28] , [29] . However, it is unclear whether MOD-1 is involved in feeding regulation. We detected expression of mod-1 in RIM and RIC interneurons ( Fig. 2e ). The functional sites of MOD-1 were further localized to the RIM and RIC neurons by reconstitution experiments in mod-1 mutants ( Fig. 2c ). The RIM and RIC neurons are among the few neurons in C. elegans that synthesize and release octopamine (OA) and tyramine (TA), biogenic amines that modulate key behaviours in both vertebrates and invertebrates [30] . In C. elegans , exogenous TA or OA inhibits egg laying and pharyngeal pumping and generally opposes the action of 5-HT [31] , [32] . It is possible that 5-HT released from NSM neurons acts through MOD-1, and suppresses the activities of RIM/RIC neurons in blocking the release of TA/OA. In mod-1 mutants, more TA/OA is released, which can then counteract the 5–HT-mediated increase in pumping. If this is true, we would expect that the response to diacetyl can be restored by lowering the TA/OA level in mod-1 mutants. Indeed, this was what we saw in mod-1;tdc-1 double mutants ( Fig. 2d ). tdc-1 encodes a tyrosine decarboxylase, which is required to convert tyrosine into TA [30] . As TA is the precursor for OA, knocking out the tdc-1 gene eliminates both TA and OA production. Diacetyl-induced feeding facilitation was not affected in tdc-1 single mutant controls. Table 1 Relative pumping rates C. elegans mutants. Full size table Circuits underlying feeding suppression However, quinine- and isoamylol-induced inhibition of pumping was completely blocked in tdc-1 mutants, whereas pumping in tbh-1 mutants was only partially inhibited ( Fig. 3a and Supplementary Fig. S10a ). tbh-1 encodes a TA β-hydroxylase required to convert TA into OA [30] . These results are consistent with the inhibitory role of TA/OA in pumping regulation [32] . 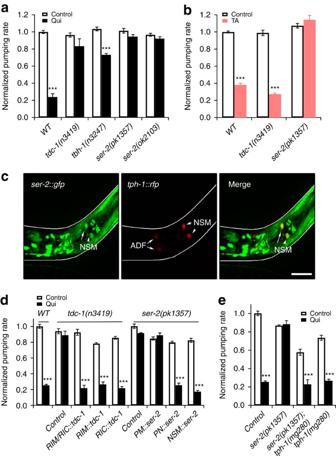Figure 3: Identification of the neurons and genes required for quinine (Qui)-induced feeding suppression. (a) Quinine-induced feeding suppression requirestdc-1andser-2, which encode an enzyme for making tyramine and a tyramine receptor, respectively.tbh-1encodes an enzyme to convert tyramine into octopamine. Normalized pumping rates for various strains under control and quinine (5 mM) stimulation conditions are shown. (b) TDC-1 acts upstream of tyramine release, whereas SER-2 acts downstream of tyramine. Tyramine (2 mM, TA) was applied exogenously. (c) Expression patterns ofser-2andtph-1. SER-2 and TPH-1 are coexpressed in NSM neurons. Scale bar, 20 μm. (d) Neuron-specific transgene rescue experiments localize the functional sites oftdc-1andser-2to RIM/RIC and NSM neurons, respectively. Promoters used werePtdc−1for RIM/RIC,Pgcy−13for RIM,Ptbh−1for RIC,Pmyo−2for pharyngeal muscles (PM),Pglr−7for pharyngeal neurons (PNs),Ptph−1for NSM. (e) The loss-of-inhibition phenotype ofser-2mutants is suppressed by eliminating serotonin intph-1mutants.tph-1itself is not required for quinine-induced feeding suppression. The feeding rates of N2 animals used for normalization ina,b,d,ewere 243, 256, 248 and 248 pumps per min, respectively. Statistics (a,b,d,e): ***P<0.001 (Student'st-test). Data are averaged from 10 to 12 animals for each condition. Error bars represent s.e.m. WT, wild type. Figure 3: Identification of the neurons and genes required for quinine (Qui)-induced feeding suppression. ( a ) Quinine-induced feeding suppression requires tdc-1 and ser-2 , which encode an enzyme for making tyramine and a tyramine receptor, respectively. tbh-1 encodes an enzyme to convert tyramine into octopamine. Normalized pumping rates for various strains under control and quinine (5 mM) stimulation conditions are shown. ( b ) TDC-1 acts upstream of tyramine release, whereas SER-2 acts downstream of tyramine. Tyramine (2 mM, TA) was applied exogenously. ( c ) Expression patterns of ser-2 and tph-1 . SER-2 and TPH-1 are coexpressed in NSM neurons. Scale bar, 20 μm. ( d ) Neuron-specific transgene rescue experiments localize the functional sites of tdc-1 and ser-2 to RIM/RIC and NSM neurons, respectively. Promoters used were P tdc−1 for RIM/RIC, P gcy−13 for RIM, P tbh−1 for RIC, P myo−2 for pharyngeal muscles (PM), P glr−7 for pharyngeal neurons (PNs), P tph−1 for NSM. ( e ) The loss-of-inhibition phenotype of ser-2 mutants is suppressed by eliminating serotonin in tph-1 mutants. tph-1 itself is not required for quinine-induced feeding suppression. The feeding rates of N2 animals used for normalization in a , b , d , e were 243, 256, 248 and 248 pumps per min, respectively. Statistics ( a , b , d , e ): *** P <0.001 (Student's t -test). Data are averaged from 10 to 12 animals for each condition. Error bars represent s.e.m. WT, wild type. Full size image We found ser-2 , which encodes a TA receptor [33] , [34] , to be another interesting gene involved in ASH-mediated pumping inhibition ( Fig. 3a , Table 1 ). In ser-2 mutants, all quinine-, isoamylol- and TA-mediated feeding suppression was blocked ( Fig. 3a,b and Supplementary Fig. S10 ). Exogenous application of both TA and OA suppressed feeding to a similar extent in N2 and tdc-1 mutants, and this feeding suppression was blocked in ser-2 mutants ( Fig. 3b and Supplementary Fig. S11 ). It is thus likely that TA and OA act redundantly in mediating feeding suppression and that SER-2 acts downstream of TA/OA. SER-2 is widely expressed in a set of sensory, inter- and motor-neurons, for example, AIY, AIZ and RIA, as well as in pharyngeal NSM cells and head muscles [35] . We confirmed that ser-2 is expressed in NSM neurons and co-localizes with tph-1 ( Fig. 3c ). Reconstitution of SER-2 in NSM neurons, but not in pharyngeal muscles, rescued the loss of inhibition phenotype of ser-2 mutants ( Fig. 3d ), suggesting that SER-2 acts in NSM neurons. We verified that TA/OA is released from RIM/RIC neurons as reconstitution of TDC-1 in RIM, RIC or both neurons in tdc-1 mutants restored the inhibitory effect of quinine ( Fig. 3d ). Hence, TA/OA released from RIM/RIC neurons is likely to inhibit 5-HT release from the NSM via acting on SER-2. In the absence of SER-2, release of 5-HT is not negatively controlled. Excessive 5-HT acts on MOD-1 and inhibits the release of TA/OA from RIM/RIC neurons, thus blocking signalling through RIM/RIC neurons during the feeding suppression induced by ASH sensory neurons. If this is true, the loss of inhibition phenotype of ser-2 should be rescued simply by removing 5-HT. Indeed, in ser-2;tph-1 double mutants, both quinine and isoamylol were able to induce inhibition of pumping, as in wild-type animals ( Fig. 3e and Supplementary Fig. S10b ). In tph-1 single mutants, as expected, although pumping rates were lower than those of wild-type animals (apparently due to the lack of 5-HT), they could be further reduced by quinine or isoamylol. Reciprocal inhibition between NSM and RIM/RIC neurons Our data indicate that NSM and RIM/RIC act as two control centres that transmit signals, 5-HT and TA/OA, that facilitate or suppress pumping rate, respectively. To provide further functional evidence, we expressed the Ca 2+ -sensitive fluorescent protein G-CaMP2.0 (ref. 36 ) in NSM and RIM/RIC neurons and measured their Ca 2+ levels under various conditions. NSM neurons demonstrated a significant and fast decrease in Ca 2+ levels on quinine treatment, whereas diacetyl increased Ca 2+ levels in NSM neurons ( Fig. 4a,b ). In RIM neurons, we observed the exact opposite: Ca 2+ levels were increased by quinine but were inhibited by diacetyl ( Fig. 4c,d ). The time course of Ca 2+ dynamics ( Fig. 4a,c ) correlates with the behaviour change in Fig. 1c . The ability of diacetyl to inhibit RIM Ca 2+ levels was abolished in tph-1 and mod-1 mutants and could be rescued by expressing TPH-1 in NSM neurons in tph-1 mutants, or by expressing MOD-1 in RIM/RIC neurons in mod-1 mutants ( Fig. 4e ). These results are in agreement with our genetic data, which indicates that diacetyl-induced inhibition of RIM/RIC neurons requires 5-HT release from NSM neurons and subsequent activation of MOD-1 in RIM/RIC neurons. Quinine- or isoamylol-induced inhibition of Ca 2+ levels in NSM neurons was absent in tdc-1 and ser-2 mutants ( Fig. 4f and Supplementary Fig. S12 ). This could be rescued by reconstitution of TDC-1 in RIM/RIC neurons in tdc-1 mutants or SER-2 in NSM neurons in ser-2 mutants ( Fig. 4f ). These results confirm our notion that quinine-induced inhibition of NSM activity requires TA release from RIM/RIC neurons and activation of SER-2 in NSM neurons. 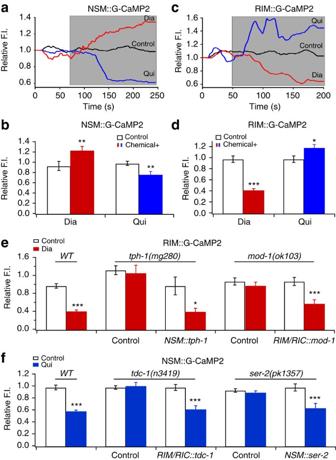Figure 4: Diacetyl and quinine oppositely regulate calcium concentration in NSM and RIM neurons. (a–d) Sample time courses and statistics of calcium levels of NSM (a,b) and RIM (c,d) neurons of freely moving animals on food in the absence (control) or the presence of 100% diacetyl (red) and 5 mM quinine (blue). Grey boxes indicate the duration of chemical application. (e) The ability of diacetyl in inhibiting the calcium levels of RIM neurons was lost intph-1andmod-1mutants, but was rescued by transgenic expression oftph-1in NSM andmod-1in RIM/RIC neurons. (f) Quinine-induced inhibition of calcium levels in NSM neurons was abolished intdc-1andser-2mutants, but was rescued by transgenic expression oftdc-1in RIM/RIC andser-2in NSM neurons. Promoters used werePtdc−1for RIM/RIC,Ptph−1for NSM. Statistics (b,d–f): *P<0.05, **P<0.01 and ***P<0.001 (Student'st-test). Data are averaged from 10 to 12 animals for each condition. Error bars represent s.e.m. Dia, diacetyl; Qui, quinine; WT, wild type. F.I., Fluorescence Intensity. Figure 4: Diacetyl and quinine oppositely regulate calcium concentration in NSM and RIM neurons. ( a – d ) Sample time courses and statistics of calcium levels of NSM ( a , b ) and RIM ( c , d ) neurons of freely moving animals on food in the absence (control) or the presence of 100% diacetyl (red) and 5 mM quinine (blue). Grey boxes indicate the duration of chemical application. ( e ) The ability of diacetyl in inhibiting the calcium levels of RIM neurons was lost in tph-1 and mod-1 mutants, but was rescued by transgenic expression of tph-1 in NSM and mod-1 in RIM/RIC neurons. ( f ) Quinine-induced inhibition of calcium levels in NSM neurons was abolished in tdc-1 and ser-2 mutants, but was rescued by transgenic expression of tdc-1 in RIM/RIC and ser-2 in NSM neurons. Promoters used were P tdc−1 for RIM/RIC, P tph−1 for NSM. Statistics ( b , d – f ): * P <0.05, ** P <0.01 and *** P <0.001 (Student's t -test). Data are averaged from 10 to 12 animals for each condition. Error bars represent s.e.m. Dia, diacetyl; Qui, quinine; WT, wild type. F.I., Fluorescence Intensity. Full size image 'Winner takes all' feature of a central integration circuit Taken together, our data reveal a central integration circuit ( Fig. 5a ), that integrates cross-modal sensory inputs and regulates feeding in a nonlinear fashion. The main integration sites were mapped to the NSM and RIM/RIC neurons. Interestingly, these neurons have neurosecretory roles. They release 5-HT and TA/OA, two opposing neurotransmitters (or neuromodulators) that can cross-inhibit each other. As there is no synaptic connection between NSM and RIM/RIC neurons, the functions of 5-HT and TA/OA here are analogous to hormones acting in the central nervous systems of higher organisms. Once a 'pleasant smell' is sensed by AWA neurons, a GLR-7-dependent relay circuit will transmit the signal to NSM neurons. This will trigger 5-HT release from the NSM neurons, which will inhibit TA/OA release from RIM/RIC neurons via MOD-1. Less TA/OA release will, in turn, relieve the inhibition of NSM neurons via SER-2 and ensure that more 5-HT is released. On the other hand, if a 'bad taste' is sensed by ASH neurons, the circuit will work in the opposite direction, favouring the maximum release of TA/OA and minimizing 5-HT release. This kind of negative-negative feedback between two signalling pathways shares a striking similarity with the 'flip-flop' circuit that is widely used in computers ( Fig. 5b ). The most striking feature of the flip-flop circuit is that it can rapidly switch between two stable states, depending on the relative strengths of the two inputs (a feature also called 'winner takes all'). To confirm this prediction from the model, we asked what would happen if we simultaneously challenged worms with two contradictory sensory inputs. As shown in Fig. 5c , when we fixed the diacetyl stimulus and scanned different concentrations of quinine, we observed a steep reversal of states, from feeding facilitation to suppression, within a narrow concentration range of quinine (2–6 mM, threefold difference). The apparent equal strengths of stimuli between diacetyl and quinine are 10% and 2.53 mM, respectively. When we unwired the integration between NSM and RIM/RIC neurons by knocking out both mod-1 and ser-2 genes, we observed a more linear response in the pumping rate within a much broader range of quinine concentrations (0.1–20 mM, 200-fold difference). The remaining linear response in the mod-1;ser-2 double mutants was possibly due to a peripheral integration mechanism downstream of NSM and RIM/RIC neurons (see Fig. 5a ). The same phenomenon was observed when we fixed the concentration of quinine at 1 mM and scanned different concentrations of diacetyl ( Fig. 5d ). In the mod-1;ser-2 double mutants lacking the ability to inhibit TA/OA release by 5-HT, even the highest concentration (100%) of diacetyl could not reverse the pumping rate to the rate observed in wild-type animals. This result indicates that the dynamic strength of these two sensory inputs in feeding modulation is different, that is, TA/OA is more potent in inhibiting the pumping rate than 5-HT. Without the 'flip-flop' circuit, 5-HT would never be able to win over TA/OA when the concentration of TA/OA is high. 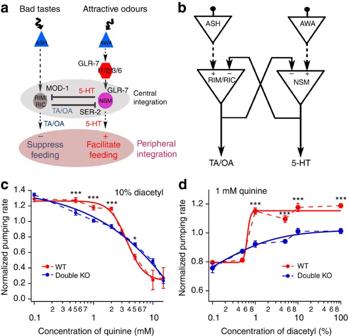Figure 5: Schematic representation of a 'flip-flop' circuit in feeding regulation and testing predictions based on the circuit. (a) Connection between neurons and the sites ofglr-7,mod-1andser-2expression. Arrows represent direct connections between neurons, whereas dashed lines indicate indirect connections. The central integration and peripheral integration sites are indicated in the grey elliptical areas. (b) Comparison of the central integration circuit inawith the electronic 'flip-flop' circuit. (c,d) Pumping rates of wild-type (WT) andmod-1(ok103);ser-2(pk1357)double mutants at different concentrations of diacetyl and quinine. Unwiring the integration at NSM and RIM/RIC neurons rendered the cross-model sensory integration from bistable nonlinear (WT) to linear responses (double mutants). All traces were fitted with the Hill equation (superimposed smooth lines). The feeding rate of N2 animals used for normalization inc,dwas 250 pumps per min. Statistics (c,d): *P<0.05 and ***P<0.001 (Student'st-test). Data are averaged from 10 to 12 animals for each condition. Error bars represent s.e.m. KO, knock out. Figure 5: Schematic representation of a 'flip-flop' circuit in feeding regulation and testing predictions based on the circuit. ( a ) Connection between neurons and the sites of glr-7 , mod-1 and ser-2 expression. Arrows represent direct connections between neurons, whereas dashed lines indicate indirect connections. The central integration and peripheral integration sites are indicated in the grey elliptical areas. ( b ) Comparison of the central integration circuit in a with the electronic 'flip-flop' circuit. ( c , d ) Pumping rates of wild-type (WT) and mod-1(ok103);ser-2(pk1357) double mutants at different concentrations of diacetyl and quinine. Unwiring the integration at NSM and RIM/RIC neurons rendered the cross-model sensory integration from bistable nonlinear (WT) to linear responses (double mutants). All traces were fitted with the Hill equation (superimposed smooth lines). The feeding rate of N2 animals used for normalization in c , d was 250 pumps per min. Statistics ( c , d ): * P <0.05 and *** P <0.001 (Student's t -test). Data are averaged from 10 to 12 animals for each condition. Error bars represent s.e.m. KO, knock out. Full size image Our appetite can be regulated by the appearance, smell and taste of food. Interestingly, some delicacies have terrible smells, for example, the famous Chinese 'smelly Tofu' or French 'smelly cheese'. Most people refuse to try them for the first time without encouragement from their surrounding company. However, once tried, most of them will love these foods for the rest of their lives, regardless of their unpleasant smell. The molecular mechanism of this and other type(s) of feeding behaviour when facing contradictory sensory stimuli has been unclear. It is likely that sensory inputs can be integrated at multiple levels to regulate feeding behaviour. In this study we demonstrate that sensory integration can happen at both the central and peripheral levels in C. elegans . The central integration circuit receives inputs from different sensory modalities in such a way that neurons sensing attractive inputs, that is, AWA and AWC neurons, are linked to NSM neurons, and neurons sensing repellents, that is ASH neurons, transmit signals to RIM/RIC neurons. The outputs of the central integration circuit are two kinds of hormones with opposing effects, 5-HT and TA/OA, released from NSM and RIM/RIC neurons, respectively. Interestingly, these two kinds of hormones cross-inhibit each other within the central integration circuit, thus generating a nonlinear, bistable output. Without this central flip-flop circuit, different sensory inputs would likely be summed linearly (that is, in mod-1;ser-2 double mutants) at the peripheral sites. The exact molecular mechanism of peripheral integration remains to be shown, and may involve unidentified receptors or even the redundant action of known receptors in pharyngeal motor neurons and/or muscles. It should be noted that the central integration circuit works in the presence of food, when animals are already receiving a variety of different sensory inputs. It is thus likely that the components of this feeding modulation system are tonically activated. As feeding regulation is fundamental to animal survival, we speculate that the basic organizational logic we have identified in C. elegans is probably converged throughout different phyla. One advantage of the flip-flop circuit is that it acts as a filter between the noisy environmental factors and the animal body, eliminating non-sense stimuli and enhancing essential stimuli. Owing to the flip-flop circuit, animals can generate a relatively stable endocrine system and behaviour in a complex and varied environment. Further studies should demonstrate whether other contradictory stimuli or other species act in the same way to regulate behaviour or metabolism. The flip-flop circuit was first invented in 1919 by Eccles and Jordan [37] , whereas simple animals as C. elegans originated the same design 80 million years ahead of human beings. Like C. elegans , human feeding is also regulated by various hormones released by the hypothalamus, some of which have opposing effects [38] . It remains to be demonstrated whether cross-modal sensations are transmitted to and integrated in the hypothalamus through a similar 'flip-flop' circuit in mammals. It would also be interesting to exploit the 'winner takes all' feature of the 'flip-flop' circuit in the fine-tuning of feeding behaviour under certain conditions, such as diet restriction or anorexia. Strains C. elegans strains were cultured on nematode growth media (NGM) plates at 20 °C, using OP50 E. coli bacterial as food resources according to standard methods [39] . Strains were obtained from the CGC ( http://www.cbs.umn.edu/CGC/ ) and the National Bio-Resources Project ( http://www.shigen.nig.ac.jp/c.elegans/index.jsp ). Strains used or generated in this study are listed in Supplementary Table S1 . Double- and triple-mutant animals with desired combination of mutations were confirmed by PCR and sequencing. All transgenic strains were generated using published methods [40] . Plasmids were injected at 50 ng μl −1 together with unc-122::rfp (20 ng μl −1 ) as coinjection marker, unless otherwise indicated. At least three independent lines were tested for each rescue experiment. Molecular biology Gateway technology was used to make the constructs. The GFP coding sequence of vector pPD95.75 (a gift from A. Fire) was replaced by the G-CaMP 2.0, TagRFP-T or C. elegans tdc-1 genes to generate a series of modified vectors. An attP1-ccdB-CmR-attP2 cassette was PCR amplified from pDONR221 (Invitrogen) with oligos that contained either Hin dIII or Age I restriction sites. The PCR fragment was then gel purified and subcloned into the unique Hin dIII and Age I sites of pPD95.75 and the other modified vectors mentioned above to obtain the modified gateway donor vectors. The promoters of tph-1, tdc-1, gcy-13, tbh-1 and mod-1 were PCR-amplified from N2 genomic DNA using primers containing attB1 and attB2 tails. These PCR fragments were recombined with the attP1 and attP2 sites in the modified donor vectors using the BP recombination reaction. In this way, P tph−1 ::G-CaMP2.0 , P tdc−1 :: G-CaMP2.0 , P tph−1 ::GFP , P tdc−1 ::GFP , P mod−1 ::TagRFP-T , P gcy−13 ::tdc-1 and P tbh−1 ::tdc-1 plasmids were generated. The promoter lengths of tph-1, tdc-1, gcy-13, mod-1 and tbh-1 are 4.5, 4.4, 2.3, 5.5 and 4.6 kb, respectively. To construct the P tph−1 ::ser-2 plasmid, the cDNA sequence of the C. elegans ser-2 gene was subcloned into the Sal I and Kpn I sites of vector pPD49.26 (a gift from A. Fire). The tph-1 promoter was then inserted between the Sph I and Sal I sites of the vector. To construct the P tdc−1 ::mod-1 plasmid, a 4,073-bp genomic DNA fragment including all introns and exons of mod-1 was PCR-amplified from N2 genomic DNA and subcloned into the Nhe I and Kpn I sites of vector pPD49.26. The tdc-1 promoter was then inserted between the Bam HI and Nhe I sites of the vector. To construct the P tph−1 ::glr -7 plasmid, a 3,657-bp genomic DNA fragment including all the introns and exons of glr-7 was PCR-amplified from N2 genomic DNA and subcloned into the Nhe I and Kpn I sites of pPD49.26. The tph-1 promoter was inserted into the Msc I and Nhe I sites of the vector. Behavioural assays All behavioural assays were performed on young adults. To assay pumping rate, we measured the time required to complete 20 pumps. Four to six measurements were recorded for every animal, and at least 8–12 animals were tested per experiment, with all experiments being repeated at least three times. To test the effect of various volatile chemicals on the modulation of feeding, well-fed young adult worms were transferred to new plates seeded with OP50. After 10 min, 2 μl of volatile chemicals (diacetyl or isoamylol, all from Sigma) was added to the lid, and the plate was sealed for 5 min before recording the pumping rate. Serotonin, TA and OA were dissolved in M9 buffer and spread on the NGM plates with food at a final concentration of 2 mM. Quinine was dissolved in M9 buffer at a concentration of 5 mM and applied to the NGM plates. Young adults were transferred to these NGM plates after 2 h, and the number of pumps was counted after 5 min for 10 min. For the control, M9 buffer was added to the plates. Avoidance of 100% isoamylol was measured as described previously [5] with slight modifications: well-fed animals were transferred to plates with food for 10 min. Then, a pulled glass electrode with a 1 MΩ resistance was dipped in 100% isoamylol and placed in front of the nose of a forward-moving animal for 2 s. The response of single animals within 4 s was recorded as either a positive (backward movement) or negative (no backward movement) response. The locomotion assay used here was based on that used in a previous study [41] . Briefly, control animals and chemical-exposed animals were transferred to plates without food. After 10 min, the number of front body bends within 20-s intervals was counted for a period of 5 min. Fluorescence imaging Fluorescence images of G-CaMP2.0 were taken under a Zeiss Discovery V8 fluorescent microscope with a ×20 objective lens. Young adult worms expressing G-CaMP2.0 in NSM or RIM/RIC neurons were transferred to new NGM plates seeded with OP50. A hole was cut in the lid and covered with a 25-mm 00# coverslip, to which 2 μl volatile chemicals was added. Quinine was added directly to the agar plate. The plates were then sealed and images of cell bodies were taken after 5 min of chemical stimulation when pumping rates had already been increased (by diacetyl) or decreased (by isoamylol or quinine). An inverted Olympus IX81 fluorescent microscope equipped with a ×20, NA0.75 objective lens was used to measure the time course of Ca 2+ . To keep the neuron of a moving worm within the field of view of the charge-coupled device, we used the PhotoTrack system from Applied Scientific Instrumentation (ASI, Eugene, USA) combined with ASI's closedloop XY stages [42] . With the help of the PhotoTrack system, the G-CaMP2.0 fluorescence of NSM or RIM/RIC neurons in freely moving worms was recorded with an Andor Luca EM-CCD at 2 Hz. Co-localization of tdc-1:: GFP and mod-1:: TagRFP-T or tph-1:: TagRFP-T and ser-2:: GFP was examined using an Andor Revolution XD laser confocal microscope system based on a spinning-disk confocal scanning head, CSU-X1 (Yokogawa Electric), under the control of Andor IQ 1.91 software. The confocal microscope was constructed on an Olympus IX-71 inverted microscope (Olympus, Tokyo, Japan) equipped with a ×60 objective lens (numerical aperture=1.45, Olympus, Japan). Images were displayed and analysed by Image-J 1.43b (Wayne Rasband, National Institutes of Health, USA). Data analysis Data analysis was conducted using IGOR Pro 5.01 (Wavemetrics, Portland, OR, USA). Results are presented as mean values±s.e.m. from 10 to 12 animals, unless otherwise indicated. Statistical significance was evaluated using the Student's t -test. Asterisks denote statistical significance: * P <0.05, ** P <0.01 and *** P <0.001. How to cite this article: Li, Z. et al . Dissecting a central flip-flop circuit that integrates contradictory sensory cues in C. elegans feeding regulation. Nat. Commun. 3:776 doi: 10.1038/ncomms1780 (2012).